PP2A and Aurora differentially modify Cdc13 to promote telomerase release from telomeres at G2/M phase In yeast, the initiation of telomere replication at the late S phase involves in combined actions of kinases on Cdc13, the telomere binding protein. Cdc13 recruits telomerase to telomeres through its interaction with Est1, a component of telomerase. However, how cells terminate the function of telomerase at G2/M is still elusive. Here we show that the protein phosphatase 2A (PP2A) subunit Pph22 and the yeast Aurora kinase homologue Ipl1 coordinately inhibit telomerase at G2/M by dephosphorylating and phosphorylating the telomerase recruitment domain of Cdc13, respectively. While Pph22 removes Tel1/Mec1-mediated Cdc13 phosphorylation to reduce Cdc13–Est1 interaction, Ipl1-dependent Cdc13 phosphorylation elicits dissociation of Est1– TLC1 , the template RNA component of telomerase. Failure of these regulations prevents telomerase from departing telomeres, causing perturbed telomere lengthening and prolonged M phase. Together our results demonstrate that differential and additive actions of PP2A and Aurora on Cdc13 limit telomerase action by removing active telomerase from telomeres at G2/M phase. Telomeres are dynamic DNA–protein complexes that protect the ends of linear chromosomes, prevent detrimental chromosome rearrangements and defend against genomic instability and the associated risk of cancer [1] , [2] , [3] , [4] , [5] . Telomeres, consisting of tandem repeats of short G-rich sequences, are synthesized by the enzyme telomerase [6] , [7] . The catalytic core of telomerase is composed of a reverse transcriptase and an RNA subunit. The reverse transcriptase utilizes the RNA component as a template to add the G-rich repeats onto the 3′-ends of the chromosome [6] , [7] , [8] . In budding yeast Saccharomyces cerevisiae , genes encoding components of telomerase have been identified and mutations in these genes cause a gradual loss of telomere length [9] , [10] . EST2 and TLC1 encode the reverse transcriptase catalytic protein subunit and the templating RNA, respectively [9] , [11] , [12] . In addition, the protein encoded by EST1 is associated with the RNA component of telomerase, TLC1 (refs 13 , 14 , 15 , 16 ). Other accessory factors, such as Cdc13, are required for the in vivo action of telomerase. Cdc13 is a single-stranded telomere-binding protein [17] , [18] , which forms a complex with Stn1 and Ten1. This replication protein A-like heterotrimeric complex [19] specifically binds single-strand telomeric sequences and is required for both telomere protection and telomerase recruitment [17] , [18] , [20] . It recruits telomerase to its site of action through an electrostatic interaction between Cdc13 and Est1 (refs 20 , 21 ). Some recent studies have suggested that Cdk1, Tel1 and Mec1 may phosphorylate the telomerase recruitment domain of Cdc13 to promote this Cdc13–Est1 interaction at the late S phase [22] , [23] , [24] , [25] , [26] , [27] . Most somatic cells exit G1 to stay in quiescent stage, while cancer cells actively undergo cell cycles. Cell cycle is controlled by numerous mechanisms to ensure precise DNA replication and cell division. G2/M is the stage to terminate DNA replication and execute cell division. CDK, Aurora and Polo-like kinases are three major kinases to coordinate G2/M phase progression [28] . Aurora kinases are master controllers that manage multiple processes during cell division [29] . These mitotic Ser/Thr protein kinases mediate cellular reorganization through a spatially and temporally confined pattern of phosphorylation [30] . On the other hand, mitotic exit regulation requires inactivation of mitotic kinases and activation of counteracting protein phosphatases. Protein phosphatase 2A (PP2A) phosphatases are abundant in cells and are involved in many processes, including cell growth, differentiation, apoptosis, cell motility, DNA damage response and cell cycle progression [31] . It is capable of reversing the effects of CDK-mediated positive regulation through dephosphorylating Cdc25 and Wee1 (refs 32 , 33 ). In addition, PP2A is particularly important for timely dephosphorylation of various CDK substrates during mitotic exit [34] . PP2A, thus, opposes not only CDK activation but also its activity by dephosphorylating downstream effectors to promote efficient cell cycle progression. Cdc13 binds Est1 to recruit telomerase [35] , [36] , [37] , and recent reports have suggested that the phosphorylations on the telomerase recruitment domain of Cdc13 may promote telomerase recruitment [22] , [26] , [27] . However, this proposed signalling has been controversial [38] , [39] . Here, we investigated the effects of Cdc13 phosphorylation on the Cdc13–Est1–telomerase signalling. We provided further evidence that phosphorylations of S249 and S255 of Cdc13 contribute to Est1-mediated telomerase recruitment at the late S phase. Phosphorylated S249 and S255 of Cdc13 are subsequently dephosphorylated by PP2A phosphatase and Cdc13 is phosphorylated by Aurora kinase at S314. Inactivation of these two regulations delays telomerase departure at the G2/M phase, which causes elongated telomeres and prolonged M phase. Interestingly, PP2A phosphatase and Aurora kinase use distinct mechanisms to remove telomerase from telomeres: while PP2A phosphatase alleviates the Cdc13–Est1 interaction, Aurora kinase reduces the Est1– TLC1 interaction. Therefore, cells use multiple pathways to differentially and additively remove telomerase from telomeres at the G2/M phase to terminate telomere replication. PP2A dephosphorylates Cdc13 serine 249 and 255 Previous studies imply that phosphorylation of Cdc13 may promote telomerase recruitment ( Fig. 1a ) [22] , [23] , [24] , [25] , [26] , [27] . To examine the possibility that recruitment of telomerase by Cdc13 may be repressed by phosphatases, we determined the phosphorylation level of Cdc13 throughout the cell cycle for wild type (WT) and various phosphatase deletion strains. As shown in Fig. 1b and Supplementary Fig. 1 , WT Cdc13 is hyper-phosphorylated at late S phase (40 min) and then decreased at G2/M (60–140 min) after α-factor synchronization. If Cdc13 is dephosphorylated by a phosphatase, phosphorylations should accumulate at the G2/M phase when the relevant phosphatase is eliminated. Some Tel1/Mec1 substrates were previously reported to be removed by the phosphatases Pph3, Pph21, Pph22, Ptc2 and Ptc3 (ref. 40 ). We therefore tested the Cdc13 protein mobility in these corresponding deletion strains by western blot analysis. As shown at the lower panel of Fig. 1b , Cdc13 in the pph22 strain displayed a higher mobility shift than that in WT and other phosphatase mutant strains at the 60 min time points. The deletions did not significantly perturb the steady-state levels of Cdc13 ( Fig. 1c ). These results suggest that Pph22, a catalytic subunit of PP2A, may regulate the function of Cdc13. 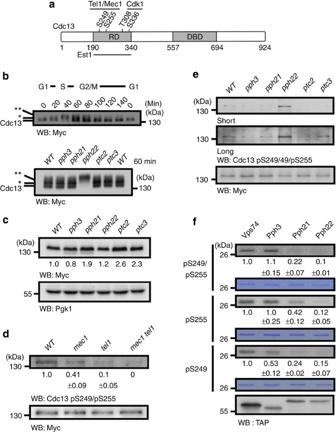Figure 1: Pph22 dephosphorylates phosphorylation of Cdc13 at Serine 249 and 255in vivoandin vitro. (a) Schematic diagram of Cdc13 illustrates its domain structure, phosphorylation sites and kinases that phosphorylate these sites. The telomerase recruitment domain (RD) and DNA-binding domain (DBD) are indicated. (b) Cell cycle-dependent phosphorylation of Cdc13. Overnight culture was grown to early log phase in YPD, arrested at G1 by α-factor, and released into cell cycle. Cells were collected at 20-min intervals for 140 min and Cdc13 was analysed by western blot analysis (WB). Cdc13 mobility in WT and different mutant strains was specifically compared at 60 and 80 min. SDS–PAGE (5%) was used to separate the hyper- and hypo-phosphorylated Cdc13, which are indicated by double (**) and single asterisk (*), respectively. (c) The steady-state levels of Cdc13 are not significantly affected in different phosphatase mutants. Endogenously expressed Cdc13 was chromosomally tagged with Myc9. Pgk1 is a loading control. (d) Endogenously expressed Cdc13 was chromosomally tagged with Myc9. Cells were nocodazole-arrested and Cdc13 was immunoprecipitated. The pS249/pS255 phospho-specific antibody detected phosphorylations were decreased inmec1,tel1andmec1 tel1mutants. (e) Western analysis of immunoprecipitated Cdc13 from nocodazole-arrested phosphatase mutants using the pS249/pS255 phospho-specific antibody. Both long and short exposures are shown. (f)In vitrophosphatase assay. Recombinant Cdc13(227–277), Cdc13-S249A(227–277) and Cdc13-S255A(227–277) were32P-labelled at S249 and S255 by Mec1. These substrates were treated with immunoprecipitants from the indicated tagged phosphatase strains. A non-phosphatase protein, Vps74, was used as a negative control. Proteins were resolved by SDS–PAGE and the phosphorylated proteins were detected by autoradiography (shown on top). The gels were also Coomassie blue stained (shown below) to confirm that samples were equally loaded. Figure 1: Pph22 dephosphorylates phosphorylation of Cdc13 at Serine 249 and 255 in vivo and in vitro . ( a ) Schematic diagram of Cdc13 illustrates its domain structure, phosphorylation sites and kinases that phosphorylate these sites. The telomerase recruitment domain (RD) and DNA-binding domain (DBD) are indicated. ( b ) Cell cycle-dependent phosphorylation of Cdc13. Overnight culture was grown to early log phase in YPD, arrested at G1 by α-factor, and released into cell cycle. Cells were collected at 20-min intervals for 140 min and Cdc13 was analysed by western blot analysis (WB). Cdc13 mobility in WT and different mutant strains was specifically compared at 60 and 80 min. SDS–PAGE (5%) was used to separate the hyper- and hypo-phosphorylated Cdc13, which are indicated by double (**) and single asterisk (*), respectively. ( c ) The steady-state levels of Cdc13 are not significantly affected in different phosphatase mutants. Endogenously expressed Cdc13 was chromosomally tagged with Myc 9 . Pgk1 is a loading control. ( d ) Endogenously expressed Cdc13 was chromosomally tagged with Myc 9 . Cells were nocodazole-arrested and Cdc13 was immunoprecipitated. The pS249/pS255 phospho-specific antibody detected phosphorylations were decreased in mec1 , tel1 and mec1 tel1 mutants. ( e ) Western analysis of immunoprecipitated Cdc13 from nocodazole-arrested phosphatase mutants using the pS249/pS255 phospho-specific antibody. Both long and short exposures are shown. ( f ) In vitro phosphatase assay. Recombinant Cdc13(227–277), Cdc13-S249A(227–277) and Cdc13-S255A(227–277) were 32 P-labelled at S249 and S255 by Mec1. These substrates were treated with immunoprecipitants from the indicated tagged phosphatase strains. A non-phosphatase protein, Vps74, was used as a negative control. Proteins were resolved by SDS–PAGE and the phosphorylated proteins were detected by autoradiography (shown on top). The gels were also Coomassie blue stained (shown below) to confirm that samples were equally loaded. Full size image Our previous study showed that Cdc13 is phosphorylated at S225, S249, S255 and S306 by Tel1 and Mec1, and that S249 and S255 are two important residues to promote telomerase recruitment [22] . To test whether Pph22 targets these two phosphorylation sites, we raised a Cdc13 S249/S255 phospho-specific polyclonal antibody and the antibody exhibited higher binding affinity to phospho-S249/S255 and phospho-S255 than phospho-S249 ( Supplementary Figs 2a, b and d ). Meanwhile, this phospho-specific antibody could detect slight phosphorylation of Cdc13-S249/S255 in cdc13-Q250/Q256A cells, suggesting that other kinases might phosphorylate Cdc13-S249/S255 ( Supplementary Fig. 2c ). As shown in Fig. 1d , this antibody could recognize endogenously expressed WT Cdc13-Myc 9 protein immunoprecipitated from nocodazole-arrested yeast cells (lane 1). Reduction of phosphorylation was clearly observed in mec1 , tel1 and mec1 tel1 mutant strains (lanes 2–4). Importantly, phosphorylation on S249/S255 accumulates in the G2/M arrested pph22 mutant ( Fig. 1e ). These data demonstrate that Pph22 can antagonize Tel1/Mec1-catalysed Cdc13 phosphorylation at pS249/pS255 in vivo . To determine whether Pph22 can directly regulate Cdc13 phosphorylation, we phosphorylated recombinant Cdc13(227–277), Cdc13-S249A(227–277) and Cdc13-S255A(227–277) by immunoprecipitated Mec1 and performed phosphatase assays with IgG-precipitated Pph22-TAP. Three IgG-precipitated tandem affinity purification (TAP) tagged proteins, Vps74, Pph3 and Pph21, were used as controls. Vps74 is required for Golgi localization of glycosyltransferases [41] ; Pph3 was reported to dephosphorylate Cdc13 pS306 (ref. 42 ); and Pph21 is another nuclear phosphatase in the PP2A complex [43] . As shown in Fig. 1f , Pph21 and Pph22 efficiently dephosphorylated Cdc13 on single phosphorylated S249 or S255, or double S249/255 phosphorylations in vitro . Pph3 only dephosphorylated phosphorylated S249, whereas Vps74 showed no phosphatase activity on Cdc13 S249/S255 phosphorylations. Therefore, in vivo and in vitro data both demonstrate that Pph22 can dephosphorylate Cdc13 at S249 and S255. Loss of PPH22 leads to delayed telomerase departure To examine how telomeric functions are affected by Pph22, we analysed the effect of pph22 mutation on telomere replication. Heterozygous pph3/PPH3 , pph21/PPH21 and pph22/PPH22 diploid strains (YPH501 background) were sporulated and dissected. The telomere length of each individual yeast colony derived from the dissected spores was measured after ~100 population doublings. Southern blot analysis showed that pph22 , but not pph3 and pph21 , mutation resulted in telomere lengthening ( Fig. 2a ), and this Pph22-mediated regulation was telomerase- and Tel1/Mec1 dependent ( Supplementary Fig. 3 ), suggesting that Tel1/Mec1 and Pph22 participate in the same pathway. Telomere shortening was observed in cdc13-S249A , cdc13-S255A and cdc13-S249/S255A cells from solid plates ( Fig. 2b,c ). In a liquid culture assay, when cultures starting from freshly dissected spores were repeatedly diluted, telomere shortening and marked telomere lengthening from survivor formation could be observed in telomerase pathway-defective strains after several dilutions [44] . Similarly, cdc13-S249/255A cells displayed gradual telomere shortening, survivor formation and cellular senescence phenotypes, and these phenotypes were recovered in cdc13-S249/255D cells ( Supplementary Fig. 4 ). All these findings indicate that phosphorylation/dephosphorylation of these two residues modulate telomerases recruitment. To further investigate whether one dephosphorylation site is more critical than the other in the Pph22-mediated function, the telomere length was analysed in spores from diploid yeast strains harbouring pph22 in combination with cdc13-S249A , cdc13-S255A or cdc13-S249/S255A . Telomere was longer in pph22 and pph22 cdc13-S249A strains than that in WT and cdc13-S249A , respectively ( Fig. 2b,c and Supplementary Fig. 5 ), but these phenotypes were eliminated in cdc13-S255A and cdc13-S249/S255A . Therefore, we conclude that dephosphorylation at Cdc13 S255 is more critical for Pph22-mediated regulation. Finally, we wish to address whether Pph22-mediated Cdc13 dephosphorylation is essential for de novo telomere addition. We tested the sudden telomere elongation by the de novo telomere addition assay ( Supplementary Fig. 6a ) [45] . Cells that were arrested by α-factor at G1 phase were released into the cell cycle and the pph22 strain displayed faster kinetics of telomere addition than WT and pph21 cells in the subsequent generations ( Supplementary Fig. 6b ). This result indicates that dephosphorylation of Cdc13 at amino acids 249 and 255 reduces de novo telomere addition. 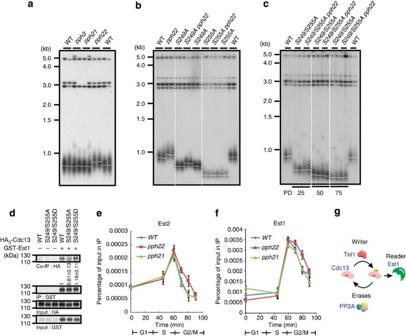Figure 2:pph22mutation results in telomere lengthening and delayed eviction of telomerase. (a) Telomere analysis ofpph21andpph22mutants. The telomere length of each individual colony derived from the dissected spore was measured at 100 generations (population doubling, PD100). (b) Telomere analysis ofpph22in WT,cdc13-S249Aandcdc13-S255Amutation backgrounds. (c) Telomere analysis ofpph22incdc13-S249/S255Abackground. Telomere length was measured at 25, 50 and 75 generations. (d) Co-IP assay indicated thatcdc13-S249/S255Amutation reduces its interaction with Est1, whereascdc13-S249/S255Dincreases. The levels of signal compared with that of the WT are shown below. (e) ChIP assays showed that cell cycle-dependent departure of Est2 at telomeres is delayed inpph22mutant compared with that in WT andpph21cells expressing Myc18-tagged Est2 (n=6,Pvalues at 70 and 80 min are <0.01, Student’st-test, two tailed). Bars, s.d. (f) ChIP assays showed that cell cycle-dependent departure of Est1 at telomeres is delayed inpph22mutant compared with that in WT andpph21cells expressing Myc18-tagged Est1 (n=6,Pvalues at 70 and 80 min are <0.01, Student’st-test, two tailed). Bars, s.d. (g) The stepwise modification on Cdc13 provides a writer-reader-eraser circuit to govern telomerase recruitment and departure. A white line marks the mean density of the autoradiographical signal ina–c. Figure 2: pph22 mutation results in telomere lengthening and delayed eviction of telomerase. ( a ) Telomere analysis of pph21 and pph22 mutants. The telomere length of each individual colony derived from the dissected spore was measured at 100 generations (population doubling, PD100). ( b ) Telomere analysis of pph22 in WT, cdc13-S249A and cdc13-S255A mutation backgrounds. ( c ) Telomere analysis of pph22 in cdc13-S249/S255A background. Telomere length was measured at 25, 50 and 75 generations. ( d ) Co-IP assay indicated that cdc13-S249/S255A mutation reduces its interaction with Est1, whereas cdc13-S249/S255D increases. The levels of signal compared with that of the WT are shown below. ( e ) ChIP assays showed that cell cycle-dependent departure of Est2 at telomeres is delayed in pph22 mutant compared with that in WT and pph21 cells expressing Myc 18 -tagged Est2 ( n =6, P values at 70 and 80 min are <0.01, Student’s t -test, two tailed). Bars, s.d. ( f ) ChIP assays showed that cell cycle-dependent departure of Est1 at telomeres is delayed in pph22 mutant compared with that in WT and pph21 cells expressing Myc 18 -tagged Est1 ( n =6, P values at 70 and 80 min are <0.01, Student’s t -test, two tailed). Bars, s.d. ( g ) The stepwise modification on Cdc13 provides a writer-reader-eraser circuit to govern telomerase recruitment and departure. A white line marks the mean density of the autoradiographical signal in a – c . Full size image Cdc13 recruits telomerase mainly through binding to a telomerase subunit Est1 to recruit the RNA subunit of telomerase, TLC1 (ref. 35 ). Since S249 and S255 lie in the Est1-interacting region [20] , [36] , [37] , we next asked whether Tel1/Mec1/Pph22-dependent phosphorylation/dephosphorylation of Cdc13 plays a role in coordinating the interaction between Cdc13 and Est1. To this end, the chromosomal copy of CDC13 and EST1 was tagged with hemagglutinin (HA 3 ) and glutatione S-transferase (GST), respectively, and expressed under the control of galactose-inducible promoters. Overexpressed GST-Est1 was precipitated by anti-GST antibodies and precipitates were detected by western blot analysis for HA 3 -Cdc13. We first verified the interaction between Cdc13 and Est1 ( Fig. 2d , lanes 1 and 4). Mutation of S249 and S255 to alanine decreased the interaction between Cdc13 and Est1 (lane 5) but mutation to phosphomimetic aspartic acid maintained the interaction (lane 6). Chromatin immunoprecipitation (ChIP) assays showed that cell cycle-dependent departures of Est2 and Est1 from telomeres were also delayed in yeast harbouring pph22 mutant compared with those in WT and pph21 strains ( Fig. 2e,f and Supplementary Figs 7 and 8 ). Since cdc13-S255A mutation caused a more prominent effect on telomere shortening, we examined whether cdc13-S255A mutation abolished the recruitment of telomerase ( Supplementary Fig. 9 ). Cell cycle-dependent recruitment of Est2 and Est1 was compromised in cdc13-S255A and cdc13-S255A pph22 cells, suggesting that the S255 phosphorylation plays a critical role in telomerase recruitment. Together, these data indicate that Pph22-dependent dephosphorylation of Cdc13 provides a negative regulation on the Cdc13–Est1 interaction and telomerase recruitment during cell cycle progression ( Fig. 2g ). Aurora phosphorylates Cdc13 serine 314 at G2/M phase After obtaining the above results, we wondered whether there are additional critical regulations that might be essential to stop telomere replication at the G2/M phase. Since multiple phosphorylations on Cdc13 promote telomerase recruitment, we surmised that distinct Cdc13 phosphorylations may also modulate telomerase departure. Using mass spectrometry (MS) to analyse phosphorylation sites of overexpressed Cdc13-Myc 9 in S. cerevisiae , we identified new phosphorylation sites S314, S324 and S333 on Cdc13 ( Fig. 3a ) that have not been well studied previously [22] , [26] , [27] , [42] ( Supplementary Fig. 10 ). We then used Southern blot analysis to examine whether these phosphorylations would affect telomere replication ( Fig. 3b ). Interestingly, an apparent telomere lengthening was observed in cdc13-S314A cells. By bioinformatic analysis, we found that S314 fits into a consensus sequence of Aurora kinase substrates ( Fig. 3c ) [46] . We thus raised a pS314-specific antibody to examine Cdc13 phosphorylation and its regulation in vivo . Western blot analysis of immunoprecipitated Cdc13-Myc 9 showed that this antibody was phospho-specific and the antibody recognized signal was abolished when immunoprecipitants was prepared from the S314A mutant ( Supplementary Fig. 11 ). Phosphorylation of S314 was largely dependent on Aurora kinase because the signal was greatly reduced in immunoprecipitants prepared from nocodazole-arrested temperature-sensitive ipl1-4 mutant following growth at non-permissive temperature ( Fig. 3c ). To identify at which cell cycle stage Cdc13 is phosphorylated, cultures synchronized with α-factor were analysed by phospho-specific antibodies. As shown in Fig. 3d , phosphorylation of S249 and S255 was detected at 40 min after release in WT but the signal accumulated from 60 to 100 min in the pph22 mutant strain. On the other hand, phosphorylation of S314 accumulated after 60 min and reached maximum at G1. Immunoprecipitation (IP) kinase assay further demonstrated that Ipl1 phoshporylates Cdc13 in vitro using recombinant Cdc13 ( Fig. 3e ). These data suggest that Ipl1 directly phosphorylates Cdc13. 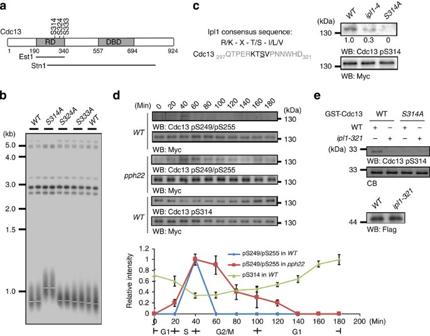Figure 3: Ipl1-mediated Cdc13 phosphorylation on S314 at M phase. (a) Schematic diagram of Cdc13 illustrates its domain structure and newly identified phosphorylation sites. The recruitment domain (RD) and DNA-binding domain (DBD) domains are indicated. (b) Telomere analysis of newly identified phosphorylation sites of Cdc13. The telomere length of individual colony derived from the dissected spore was measured at 100 population doubling (PD100). A white line marks the mean density of the autoradiographical signal. (c) The phosphorylation site of Cdc13 S314 fits into the Ipl1 consensus site (R/K-X-T/S*-I/L/V)46. Endogenously expressed Cdc13 was chromosomally tagged with Myc9. Cells were arrested by nocodazole and cultures were shifted to the non-permissive temperature of theipl1-4strain (37 °C). The pS314 phospho-specific antibody detected immunoprecipitated WT but not Cdc13-S314A mutant protein, and the signal was decreased in temperature-sensitiveipl1-4mutants. The same blot was stripped and reprobed with an anti-Myc antibody. (d) Phosphorylations of Cdc13 S249/S255 and S314 are cell cycle dependent. Phosphorylation of Cdc13 S249/S255 is enriched ~40–60 min (late S/G2) after α-factor synchronization and release. Phosphorylation of Cdc13 S314 is decreased from G1 to S phase, and enriched from M to G1 phase. α-Factor was added at 60 min again to prevent cells re-entering the next cell cycle. The quantitative analysis is shown below. Bars, s.d. (e)In vitrokinase assay was performed using immunoprecipitants of Flag-tagged Ipl1 WT or kinase-dead mutant on recombinant Cdc13(276–332). Western blot analysis was conducted using Cdc13 pS314 phospho-specific or Flag antibodies. The kinase reactions were also Coomassie blue (CB) stained (shown below) to confirm that lanes were equally loaded. Figure 3: Ipl1-mediated Cdc13 phosphorylation on S314 at M phase. ( a ) Schematic diagram of Cdc13 illustrates its domain structure and newly identified phosphorylation sites. The recruitment domain (RD) and DNA-binding domain (DBD) domains are indicated. ( b ) Telomere analysis of newly identified phosphorylation sites of Cdc13. The telomere length of individual colony derived from the dissected spore was measured at 100 population doubling (PD100). A white line marks the mean density of the autoradiographical signal. ( c ) The phosphorylation site of Cdc13 S314 fits into the Ipl1 consensus site (R/K-X-T/S*-I/L/V) [46] . Endogenously expressed Cdc13 was chromosomally tagged with Myc 9 . Cells were arrested by nocodazole and cultures were shifted to the non-permissive temperature of the ipl1-4 strain (37 °C). The pS314 phospho-specific antibody detected immunoprecipitated WT but not Cdc13-S314A mutant protein, and the signal was decreased in temperature-sensitive ipl1-4 mutants. The same blot was stripped and reprobed with an anti-Myc antibody. ( d ) Phosphorylations of Cdc13 S249/S255 and S314 are cell cycle dependent. Phosphorylation of Cdc13 S249/S255 is enriched ~40–60 min (late S/G2) after α-factor synchronization and release. Phosphorylation of Cdc13 S314 is decreased from G1 to S phase, and enriched from M to G1 phase. α-Factor was added at 60 min again to prevent cells re-entering the next cell cycle. The quantitative analysis is shown below. Bars, s.d. ( e ) In vitro kinase assay was performed using immunoprecipitants of Flag-tagged Ipl1 WT or kinase-dead mutant on recombinant Cdc13(276–332). Western blot analysis was conducted using Cdc13 pS314 phospho-specific or Flag antibodies. The kinase reactions were also Coomassie blue (CB) stained (shown below) to confirm that lanes were equally loaded. Full size image Given the fact that both S249/S255 and S314 are located at the telomerase recruitment domain, we wondered whether there is an interplay between phospho-S249/S255 and phospho-S314. Western blot analysis demonstrated that phosphorylations on S249 and S255 were only slightly altered in cdc13-S314A cells ( Supplementary Fig. 11d ). On the other hand, a 33% reduction on S314 phosphorylation was observed in cdc13-S249/S255A cells ( Supplementary Fig. 11d ). These results indicate that the phosphate groups on S249 and S255 may have an influence on the Aurora kinase-mediated S314 phosphorylation. To identify the potential cellular functions for Cdc13 S314 phosphorylation, we tested whether other telomere-related mutations would affect S314-mediated phenotypes. Telomere length was analysed in cdc13-S314 strains in combination with or without deletion of known factors involved in the telomerase pathway ( Fig. 4a–c and Supplementary Fig. 12 ). In WT and mec1 strains, single mutation serine to alanine caused telomere lengthening. These results indicate that the negative charge on this residue at a particular timing is necessary for telomere length homeostasis. Moreover, no additional or synergistic effect on telomere lengthening was observed in cdc13-S314 tel1 , cdc13-T308A-S314 and cdc13-S314 tlc1 strains. These data suggest that the S314 phosphorylation-mediated telomere regulation depends on telomerase. Besides, in the absence of Tel1/Cdk1-dependent phosphorylation on Cdc13, Ipl1-mediated phosphorylation on S314 does not modulate telomere replication. 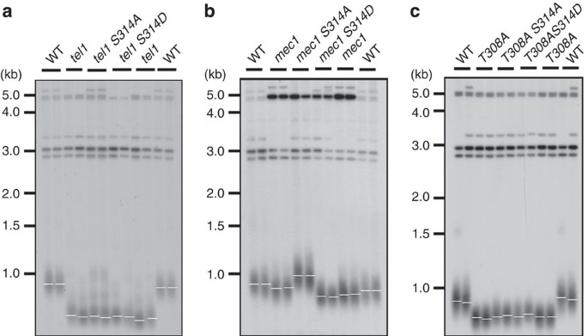Figure 4: Telomere length regulation by Cdc13 Serine 314 mutation is Tel1/Cdk1 dependent. (a) Telomere analysis of Cdc13 S314 in WT andtel1backgrounds. (b) Telomere analysis of Cdc13 S314 in WT andmec1backgrounds. A black line marks the mean density of the autoradiographical signal. (c) Telomere analysis of Cdc13 S314 in WT, andcdc13-T308Abackgrounds. A black line marks the mean density of the autoradiographical signal. A black line marks the mean density of the autoradiographical signal ina–c. Figure 4: Telomere length regulation by Cdc13 Serine 314 mutation is Tel1/Cdk1 dependent. ( a ) Telomere analysis of Cdc13 S314 in WT and tel1 backgrounds. ( b ) Telomere analysis of Cdc13 S314 in WT and mec1 backgrounds. A black line marks the mean density of the autoradiographical signal. ( c ) Telomere analysis of Cdc13 S314 in WT, and cdc13-T308A backgrounds. A black line marks the mean density of the autoradiographical signal. A black line marks the mean density of the autoradiographical signal in a – c . Full size image Aurora accelerates eviction of telomerase at G2/M phase Since serine 314 is located in the Est1- and Stn1-interacting region of Cdc13 ( Fig. 3a ) [20] , [36] , [37] , [47] , we next asked whether Ipl1-dependent phosphorylation of Cdc13 plays a role in coordinating the interaction of Cdc13 with Est1 or Stn1. When GST-Est1, GST-Stn1 and HA 3 -Cdc13 were overexpressed using galactose-inducible promoters, we detected the Cdc13–Est1 and Cdc13–Stn1 interactions. Mutation of S314 to alanine or aspartic acid did not affect the interaction of Cdc13 with Est1 or Stn1 ( Supplementary Fig. 13 ). Furthermore, mutation of S314 to alanine or aspartic acid did not affect the cell cycle-dependent departure of Est1 ( Fig. 5a ). However, cell cycle-dependent departure of Est2 from telomeres was delayed in yeast harbouring cdc13-S314A mutant compared with that in WT ( Fig. 5b and Supplementary Fig. 14 ). Mutation of S314 to alanine resulted in a twofold increase of TLC1 RNA co-immunoprecipitated with Cdc13 ( Fig. 5c ). Conversely, co-immunoprecipitated TLC1 was reduced in the cdc13-S314D mutant ( Fig. 5c ). The interaction between Est1 and TLC1 was increased in the cdc13-S314A mutant compared with that in WT ( Fig. 5d ), and co-immunoprecipitated TLC1 was reduced in the cdc13-S314D mutant ( Fig. 5d ). We could not detect a difference in Est2– TLC1 association in cdc13-S314 mutation background ( Fig. 5e ). On the other hand, cell cycle-dependent Cdc13/Est1-mediated TLC1 association was increased in yeast harbouring cdc13-S314A mutant compared with that in WT ( Fig. 5f and Supplementary Fig. 14 ). Together, these data indicate that Ipl1-dependent phosphorylation of Cdc13 plays a role to telomerase RNA departure during cell cycle progression. This regulation on telomerase departure is not through perturbing the Cdc13–Est1 interaction, but through alleviating the Est1– TLC1 interaction. 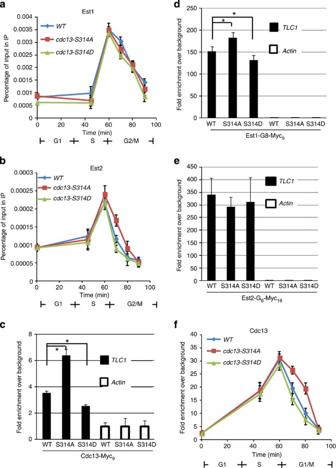Figure 5: S314 phosphorylation accelerates the departure of telomerase at M phase. (a) ChIP assays showed that cell cycle-dependent departure of Est1 at telomeres is not delayed incdc13-S314Aand incdc13-S314Dstrains (n=6,Pvalues at 70 and 80 min are >0.05, Student’st-test, two tailed). Bars, s.d. (b) ChIP assays showed that cell cycle-dependent departure of Est2 at telomeres is delayed incdc13-S314Amutant compared with that in WT andcdc13-S314Dcells expressing Myc18-tagged Est2 (n=6,Pvalues at 70 and 80 min are <0.01, Student’st-test, two tailed). Bars, s.d. (c) IP of Cdc13-Myc9from nocodazole-arrested culturein vivo. Co-immunoprecipitatedTLC1RNA was quantified by real-time reverse transcription PCR (RT–PCR). Telomerase recruitment efficiency is reduced in thecdc13-S314Dstrain (n=6,Pvalues<0.01, Student’st-test) and conversely increased in thecdc13-S314Astrain (n=6, *Pvalues<0.01, Student’st-test). Bars, s.d. (d) IP of Est1-Myc9from nocodazole-arrested culturein vivo. Co-immunoprecipitatedTLC1RNA was quantified by real-time RT–PCR. Telomerase recruitment efficiency is reduced in thecdc13-S314Dstrain (n=6,Pvalues<0.01, Student’st-test) and conversely increased in thecdc13-S314Astrain (n=6, *Pvalues<0.01, Student’st-test). Bars, s.d. (e) IP of Est2-Myc18in vivo. Co-immunoprecipitatedTLC1RNA was quantified by real-time RT–PCR. (f) IP of Cdc13-Myc9through cell cycle progressionin vivo. Co-immunoprecipitatedTLC1RNA was quantified by real-time RT–PCR.TLC1binding to Cdc13 is increased in thecdc13-S314Astrain (n=6,Pvalues at 70 and 80 min are <0.01, Student’st-test) Bars, s.d. Figure 5: S314 phosphorylation accelerates the departure of telomerase at M phase. ( a ) ChIP assays showed that cell cycle-dependent departure of Est1 at telomeres is not delayed in cdc13-S314A and in cdc13-S314D strains ( n =6, P values at 70 and 80 min are >0.05, Student’s t -test, two tailed). Bars, s.d. ( b ) ChIP assays showed that cell cycle-dependent departure of Est2 at telomeres is delayed in cdc13-S314A mutant compared with that in WT and cdc13-S314D cells expressing Myc 18 -tagged Est2 ( n =6, P values at 70 and 80 min are <0.01, Student’s t -test, two tailed). Bars, s.d. ( c ) IP of Cdc13-Myc 9 from nocodazole-arrested culture in vivo . Co-immunoprecipitated TLC1 RNA was quantified by real-time reverse transcription PCR (RT–PCR). Telomerase recruitment efficiency is reduced in the cdc13-S314D strain ( n =6, P values<0.01, Student’s t -test) and conversely increased in the cdc13-S314A strain ( n =6, * P values<0.01, Student’s t -test). Bars, s.d. ( d ) IP of Est1-Myc 9 from nocodazole-arrested culture in vivo . Co-immunoprecipitated TLC1 RNA was quantified by real-time RT–PCR. Telomerase recruitment efficiency is reduced in the cdc13-S314D strain ( n =6, P values<0.01, Student’s t -test) and conversely increased in the cdc13-S314A strain ( n =6, * P values<0.01, Student’s t -test). Bars, s.d. ( e ) IP of Est2-Myc 18 in vivo . Co-immunoprecipitated TLC1 RNA was quantified by real-time RT–PCR. ( f ) IP of Cdc13-Myc 9 through cell cycle progression in vivo . Co-immunoprecipitated TLC1 RNA was quantified by real-time RT–PCR. TLC1 binding to Cdc13 is increased in the cdc13-S314A strain ( n =6, P values at 70 and 80 min are <0.01, Student’s t -test) Bars, s.d. Full size image PP2A and Aurora act independently but additively Finally, we asked whether PP2A phosphatase and Aurora kinase work through independent pathways. Cell cycle progression and telomere length were examined in WT, single and double mutants. Additive effects in cell cycle delay and telomere lengthening were observed in the pph22 cdc13-S314A strain ( Fig. 6a,b ). These phenotypes were not observed in the pph22 ipl1-4 strain ( Supplementary Fig. 15 ), probably because Ipl1 regulates too many downstream substrates and all these regulations may engender a combinatively dominant effect on telomeres. Cell cycle-dependent departure of Est2 from telomeres was further delayed in the pph22 cdc13-S314A double mutant compared with that in pph22 and in cdc13-S314A strains ( Fig. 6c and Supplementary Fig. 7 ), as observed that Est2 binding to telomeres was 70, 34 and 44 percentage higher at the 70-min time point in pph22 cdc13-S314A , pph22 and cdc13-S314A mutants, respectively, compared with that in the WT ( Fig. 6c ). Previous studies have shown that G2/M delay alone is not sufficient to trigger telomere lengthening ( Supplementary Table 1 ), indicating an active role of Pph22 and Ipl1 in removing telomerase. These results suggest that Pph22 and Ipl1 control telomere replication through different pathways and each contributes to telomerase departure. 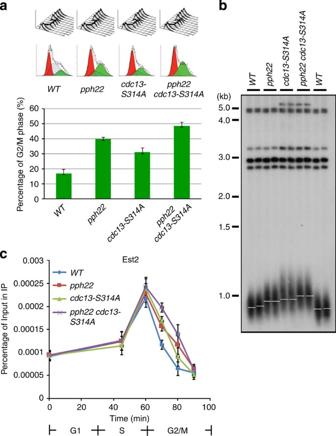Figure 6: PP2A phosphatase and Aurora kinase independently contribute to telomerase departure. (a) Delay of cell cycle inpph22 cdc13-S314Acells. Cells were α-factor synchronized and released at 30 °C. Aliquots were taken at indicated time points for flow cytometry analysis. The data at 120 min are specifically shown. Percentages of cell cycle stages were quantified according to the manufactures instructions (Becton Dickinson). Bars, s.d. (b) Telomere analysis ofpph22in the WT orcdc13-S314Abackground. Cells used in this experiment were derived from the dissected spores at 100 population doubling (PD100). A white line marks the mean density of the autoradiographical signal. (c) ChIP assays showed that cell cycle-dependent departure of Est2 at telomeres is additively delayed in thepph22 cdc13-S314Astrain compared with that in single mutants (n=6,Pvalues at 70 is <0.01,Pvalues at 80 is <0.05, Student’st-test, two tailed). Bars, s.d. Figure 6: PP2A phosphatase and Aurora kinase independently contribute to telomerase departure. ( a ) Delay of cell cycle in pph22 cdc13-S314A cells. Cells were α-factor synchronized and released at 30 °C. Aliquots were taken at indicated time points for flow cytometry analysis. The data at 120 min are specifically shown. Percentages of cell cycle stages were quantified according to the manufactures instructions (Becton Dickinson). Bars, s.d. ( b ) Telomere analysis of pph22 in the WT or cdc13-S314A background. Cells used in this experiment were derived from the dissected spores at 100 population doubling (PD100). A white line marks the mean density of the autoradiographical signal. ( c ) ChIP assays showed that cell cycle-dependent departure of Est2 at telomeres is additively delayed in the pph22 cdc13-S314A strain compared with that in single mutants ( n =6, P values at 70 is <0.01, P values at 80 is <0.05, Student’s t -test, two tailed). Bars, s.d. Full size image We previously found that Tel1 and Mec1 phosphorylate Cdc13 at S249 and S255 in vitro [22] . Several laboratories also discovered genetic and physical evidence of the importance of Tel1 in telomerase recruitment [23] , [24] , [25] . In this study, our phospho-specific antibody detected in vivo S249 and S255 phosphorylation in a Tel1/Mec1-dependent and cell cycle-dependent manner and the signal was abolished in the cdc13 S249S255A cells. Moreover, gradual telomere shortening and cellular senescence were observed in cdc13-S249/S255A cells, but partly recovered in cdc13-S249/S255D cells. All these findings suggest that the negative charges at the telomerase recruitment domain of Cdc13 facilitate the Cdc13–Est1 salt-bridge formation [26] , [48] . Contrary to expectations, a two-hybrid assay [38] found that the Cdc13 and Est1 interaction is Tel1 independent. Lack of in vivo evidence of Cdc13 S249 and S255 phosphorylation previously has caused some reasonable speculation and debate in this field. However, all these arguments are understandable and explainable. For example, the interaction between Cdc13 and Est1, as monitored by the two-hybrid assay, is S255 dependent but Tel1 independent [38] . In that case, two-hybrid assay might measure a basal level interaction between Cdc13 and Est1, and phosphorylation may stimulate their interaction in vivo only at the late S phase. However, this Tel1-mediated enhancement may not be detectable owing to the excess amounts of Cdc13 and Est1 throughout the whole-cell cycle in the two-hybrid system, which may be over the enzymatic loading for the endogenous Tel1 kinase. Here we present evidence for the first time that Cdc13 S249 and S255 are phosphorylated in vivo at the late S phase ( Fig. 3c ). Cdc13 S249 and S255 are partially phosphorylated in cdc13-Q250/Q256A mutant cells ( Supplementary Fig. 2c ), and the cdc13-Q250/Q256A mutation causes slight telomere shortening [38] . Therefore, we hypothesize that other protein kinases might phosphorylate Cdc13 S249 and S255, especially in the absence of Tel1/Mec1 kinases. The phosphorylation of Cdc13-S249/S255 is critical for telomerase recruitment and this action cannot be completely recovered by aspartate replacement in vivo . However, Cdc13-S249/S255D retains its ability to interact with Est1 in our in vitro co-IP assay. A possible explanation is that the S249/S255D mutation may bind to Est1 with the same affinity, but this binding leads to some allosteric effect on Est1– TLC1 association. Alternatively, in vitro co-IP assay using overexpressed and tagged proteins may not completely reflect the exact affinity between Cdc13 and Est1 in vivo , and Cdc13-S249/S255D does contain a little defect in Est1 binding. Our findings further strengthens the detailed mechanism of Tel1/Cdc13/Est1-mediated telomerase recruitment in S. cerevisiae [20] , [22] , [23] , [25] . The collective functions of Ccq1, Tpp1and Pot1 in Schizosaccharomyces pombe are analogous to the telomeric role of Cdc13 in S. cerevisiae [49] , [50] . Consistently, ataxia telangiectasia mutated (ATM)/ATM- and Rad3-related (ATR)-promoted Ccq1–Est1 interaction was recently revealed [51] . It will be interesting to know whether ATM/ATR promotes the TPP1–POT1 complex-mediated telomerase recruitment in mammals [52] , [53] as observed in yeasts. Adequate and timely regulation of DNA replication is critical for optimal progression of cell cycle. Telomere replication is facilitated by Cdk1/Tel1/Mec1-mediated Cdc13 phosphorylation at late S phase [22] , [23] , [24] , [25] , [26] , [27] . G2 phase is well known as the pre-mitotic phase to prepare for M phase entry. Another critical task at G2/M is to completely terminate DNA replication. Aurora is a master G2/M phase kinase [28] , and PP2A phosphatase counteracts ATM and ATR functions in DNA damage [54] . Here we demonstrate that both PP2A phosphatase and Aurora kinase promote the termination of telomere replication through modifications on Cdc13. A recent study also identifies that S314 of Cdc13 is a phosphorylation site and this phosphorylation might provide a critical regulation in telomere replication [55] . It is interesting that PP2A phosphatase and Aurora kinase use distinct mechanisms to remove telomerase. PP2A phosphatase directly removes the phosphorylations on Cdc13 S249 and S255 to reduce the electrostatic interaction between Cdc13 and Est1. On the other hand, Aurora kinase-mediated Cdc13 phosphorylation does not disturb the Cdc13–Est1 interaction but may lead to an allosteric modulation on Est1– TLC1 interaction that dissociates telomerase RNA. It may be possible that in a single cell, PP2A phosphatase helps to remove telomerase on some telomeres, whereas Aurora kinase promotes telomerase departure on other telomeres. Compromising PP2A phosphatase- and Aurora kinase-mediated regulations trigger unnecessary telomere elongation, which should be a waste of energy and lead to cell cycle delay. Moreover, although at G1 phase Aurora kinase-mediated S314 phosphorylation may provide an inhibitory effect on the Cdc13–Est1– TLC1 interaction, as previously suggested [56] at G1 phase the telomerase complex may be further recruited by the Ku complex. We previously identified that Cdk1-mediated Cdc13 phosphorylation also controls the stability of Cdc13 (ref. 27 ). This kind of modulation may send a signal for the AAA ATPase Cdc48-facilitated Cdc13 degradation [57] . Sequential phosphorylation and dephosphorylation on Cdc13 therefore offer a great platform to modulate telomerase function in vivo . Moreover, Pif1 helicase is a negative regulator of telomere replication [58] . Its helicase function facilitates cells to remove telomerase RNA from telomeres [59] . All these regulations may additively contribute to telomerase departure and serve as gatekeepers to maintain efficient cell cycle ( Fig. 7 ), and our findings provide evidence that not only initiation but also termination of telomerase recruitment plays an important role in telomere maintenance and cell cycle progression. 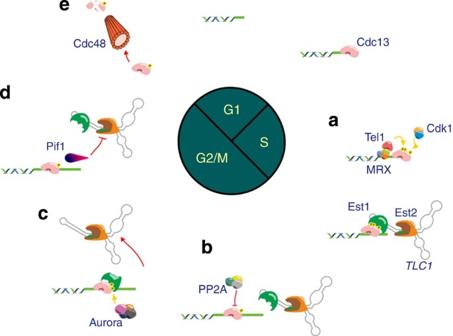Figure 7: Schematic model of PP2A phosphatase and Aurora kinase-promoted telomerase departure. (a) Cdc13 is phosphorylated by Cdk1, Tel1 and Mec1 at late S phase to recruit Est1 and the telomerase complex. (b) Pph22 dephosphorylates Cdc13 and dissociates Est1 to promote the departure of the telomerase complex. (c) Ipl1 phosphorylates Cdc13 serine 314. It may lead to an allosteric modulation on Est1–TLC1interaction that dissociates telomerase from telomeres. (d) Pif1 helicase removes telomerase RNA from telomeres59. (e) Cdk1 and AAA ATPase Cdc48 (ref.57) facilitate Cdc13 degradation. Pathwaysb–dmay occur on different telomeres to completely inactivate telomerase recruitment at M phase. Figure 7: Schematic model of PP2A phosphatase and Aurora kinase-promoted telomerase departure. ( a ) Cdc13 is phosphorylated by Cdk1, Tel1 and Mec1 at late S phase to recruit Est1 and the telomerase complex. ( b ) Pph22 dephosphorylates Cdc13 and dissociates Est1 to promote the departure of the telomerase complex. ( c ) Ipl1 phosphorylates Cdc13 serine 314. It may lead to an allosteric modulation on Est1– TLC1 interaction that dissociates telomerase from telomeres. ( d ) Pif1 helicase removes telomerase RNA from telomeres [59] . ( e ) Cdk1 and AAA ATPase Cdc48 (ref. 57 ) facilitate Cdc13 degradation. Pathways b – d may occur on different telomeres to completely inactivate telomerase recruitment at M phase. Full size image Strains and plasmids All yeast operations were performed by standard methods [60] . Strains and plasmids used in this study are listed in Supplementary Tables 2 and 3 . Mutant strains pph3Δ, pph21Δ and pph22Δ are isogenic to BY4741 ( MATa his2Δ1 leu2Δ0 met15Δ0 ura3Δ0 ) and were obtained from yeast deletion library (Invitrogen, 95401.H2). The yeast strains carrying tlc1 , mec1 , sml1 , tel1 , cdc13 and CDC13 -Myc 9 are isogenic to YPH499 ( MATa ura3-52 lys2-801_amber ade2-101_ochre trp1-Δ63 his3-Δ200 leu2-Δ1 ) (ref. 61 ). ipl1-4 is isogenic to Y300 ( MATa trp1-1 ura3-1 his3-11,15 leu2-3,112 ade2-1 can1-100) . PPH3 -TAP, PPH21 -TAP and PPH22 -TAP are isogenic to W303 ( MATa leu2-3,112 trp1-1 can1-100 ura3-1 ade2-1 his3-11,15 ). pRS304 CDC13 -Myc 9 was obtained from Dr Virginia Zakian [37] and pRS306 CDC13 was constructed by PCR containing the CDC13 open read frame and the downstream 200 nucleotides. Point mutations were introduced into CDC13 using QuickChange site-directed mutagenesis (Stratagene). To generate chromosomal cdc13 mutants, pRS306 cdc13 mutants were XhoI-digested and transformed into CDC13 strains, and the URA3 pop-out mutants were selected from the 5-fluoroorotic acid (5-FOA)-resistant colonies using PCR analysis. The ipl1-4 strain was constructed by a recombination-mediated two-step gene replacement procedure [62] , replacing the IPL1 with the ipll-4 mutant allele of pCC321. The pph22 ::KanMX4 and pph22 :: HIS3 mutants were constructed by transforming pph22 ::KanMX4 and pph22 :: HIS3 PCR fragments, respectively, into the strains. Plasmids pGEX-4T-Cdc13(227–277) were constructed by ligating a PCR product containing amino acids 227–277 of Cdc13 from pRS314 CDC13 into BamHI- and SalI-treated pGEX-4T. Plasmids pGEX-4T-Cdc13(276–332) were constructed by ligating a PCR product containing amino acids 276–332 of Cdc13 from pRS314 CDC13 into BamHI- and XhoI-treated pGEX-4T. Plasmid pYES2-Cdc13-Myc 9 was constructed by ligation of a PCR product from pRS314Cdc13-Myc 9 into KpnI-Klenow-treated pYES2. All primer sequences for PCR and mutagenesis are provided in Supplementary Table 4 . Gel electrophoresis and western blot analysis Cells were grown at 30 °C in yeast extract peptone dextrose (YPD) broth. Cell lysates were prepared with lysis buffer (150 mM NaCl, 1% Nonidet P-40, 1% deoxycholate, 0.1% SDS, 50 mM Tris–HCl, pH 7.5, and protease inhibitors) or trichloroacetic acid (TCA) precipitated [63] . Whole proteins were extracted and resolved by 10% (except Fig. 1b ) SDS–polyacrylamide gel electrophoresis (SDS–PAGE). For the supershift of Cdc13 phosphorylations, SDS–PAGE was performed by Bio-Rad PROTEIN II System. Myc 9 -tagged Cdc13 protein was detected by an anti-Myc antibody (Roche, working condition 1: 2,000). HA-tagged Cdc13 protein was detected by an anti-Myc antibody (Covance, working condition 1:2,000). GST-tagged overexpressed Cdc13, Est1 and Stn1 were detected by an anti-GST antibody (Roche, working condition 1:3,000). TAP-tagged phosphatase Pph3, Pph21 and Pph22 were detected by an anti-TAP antibody (Thermo Fisher Scientific, working condition 1:3,000). FLAG-tagged Ipl1 was detected by an anti-FLAG antibody (Sigma, working condition 1:1,000). Affinity-purified rabbit anti-Cdc13 pS249/pS255 and pS314 phospho-specific antibodies (raised against phosphopeptides SGSGYIESpQNEFNSpQLMC and TPERKTSpVPNNWHC, respectively) were used to detect phosphorylations. A cysteine residue was added to the C terminus to facilitate conjugation with a carrier protein for greater immunogenicity. To generate antibodies, rabbits were boosted with carrier-conjugated phosphopeptides once per month. Pre-immune serums were collected before boost. Injection was conducted every 4 weeks and blood samples were collected every 2 weeks. Blood samples were incubated at 37 °C for 30 min, and serum and blood cells were separated via high-speed centrifugation. Clarified serum was incubated at 56 °C for 30 min to remove complements. The specificity of antibodies was verified by means of peptide dot blot analysis. Images were captured and quantified by a bioluminescence imaging system (UVP BioSpectrum AC Imagine System, UVP). Uncropped plots are provided in Supplementary Fig. 16 . IP and co-IP IP of Cdc13-Myc 9 was conducted by 9E10 monoclonal antibodies (Roche). GST-Est1 and GST-Stn1 were immunoprecipitated by 2 μg of a GST antibody (GE). Immunoprecipitated GST-Est1 and GST-Stn1were detected by the same GST antibody (GE, working condition 1:3,000) and co-immunoprecipitated HA 3 -Cdc13 was detected by an HA antibody (Covance, working condition 1:2,000). Images were captured and quantified by a bioluminescence imaging system (UVP BioSpectrum AC Imagine System, UVP). Dot blot analysis A quantity of 50 ng of the phosphorylated or unphosphorylated peptides were spotted on nitrocellulose membranes. Dot blot analysis was conducted by standard protocol using phospho-specific antibodies. In vitro phosphatase assay In vitro phosphatase experiments were conducted using affinity-purified TAP-tagged Vps74, Pph3, Pph21 and Pph22 complexes. Recombinant Cdc13 substrates Cdc13(227–277), Cdc13-S249A(227–277) and Cdc13-S255A(227–277) were purified and pre-phosphorylated by immunoprecipitated Mec1 kinase. The kinase assay was initiated in 40 μl of kinase buffer by the addition of 10 mCi [γ‐ 32 P]ATP (3,000 Ci mmol −1 , Amersham Pharmacia Biotech), substrate (2 μg of recombinant Cdc13) and ATP to 100 μM (ref. 22 ). In vitro phosphatase experiments used affinity-purified, TAP-tagged Pph3, Pph21 or Pph22 complexes. The immunopurified phosphatase [64] were incubated with recombinant Cdc13 proteins previously created in vitro by phosphorylating with Mec1 kinase. Sample buffer (2 × ) was added, and reactions were separated by 10% SDS–PAGE and subjected to autoradiography using an X-ray film. Images were captured and quantified by a bioluminescence imaging system (UVP BioSpectrum AC Imagine System, UVP). Southern blot analysis and telomere length measurement When DNA was examined from individual colonies, the colony was expanded in 2 ml of liquid medium to obtain enough DNA for Southern analysis [65] . Genomic DNAs were digested with KpnI, separated by 1.2% agarose gel electrophoresis, and transferred to Genescreen Plus membrane (PerkinElmer). The blot was probed by a 341-bp 32 P-labelled (Invitrogen) XhoI-KpnI fragment from the 3′-end of Y′ element. Spore cells were serially diluted into or restreaked onto YPD medium. Liquid cultures were generated by inoculating spore colonies from the tetrad plate into 10 ml of liquid YEPD medium. Cultures were diluted repeatedly 1:10,000 into fresh medium at 48 or 72 h (refs 22 , 65 ). Genomic DNAs were digested with XhoI, separated by 1% agarose gel electrophoresis and transferred to Genescreen Plus membrane (PerkinElmer). The blot was probed by a 550-bp 32 P-labelled (Invitrogen) EcoRI fragment of TG 1–3 sequence. De novo telomere addition assay De novo telomere addition assay was performed as previously described [45] . UCC5706 strain was kindly provided by Dr Daniel Gottschling. The pph21 ::KanMX4 and pph22 :: Kan MX4 mutants were constructed by transforming pph21 ::KanMX4 and pph22 :: Kan MX4 PCR fragments, respectively, into UCC5706. Equal number of cells was collected for DNA preparation, enzyme digestion and Southern blot analysis. Chromatin IP ChIP analysis was performed as described [25] . In brief, cells were grown, G1 arrested and released at 24 °C in YPD broth. After crosslinking in 1% formaldehyde, cells were lysed and sonicated. IPs were carried out with anti-Myc 9E10 (Roche) and Protein G Dynabeads (Dynal) against C-terminally Myc 18 -tagged Est2 and Est1. Both an aliquot of sonicated cleared extract (input) and the immunoprecipitated material were de-crosslinked in Tris/EDTA buffer (TE) plus 1% SDS for at least 8 h at 65 °C. Quantification of immunoprecipitated DNA was obtained by real-time PCR using SYBR Green detection (Kappa) on an Applied Biosystems HT7500 machine and software, and was expressed as percent of starting (input) material. Primers used in this study are listed in Supplementary Table 4 . In a given synchrony, samples from each time point were amplified in duplicate or triplicate to obtain an average value for each sample. In addition, each synchrony was repeated six times; the data are presented as the mean of the three or more synchronies plus or minus s.d.’s. Where applicable, a two-tailed Student’s t -test was used to determine statistical significance ( P value ≤0.05) Cell cycle analysis of ChIP samples For ChIP assay, cells were grown at 30 °C in raffinose and arrested by α-factor. Galactose was added for an additional 3 h. Cells were then transferred to glucose medium with α-factor for 15 min before the α-factor was removed by centrifugation. Cells were released into cell cycle at 24 °C by the addition of protease. Samples were taken at 0, 45, 60, 70, 80 and 90 min, and were processed for fluorescence-activated cell sorting and ChIP analyses. MS analysis In order to identify the phosphorylation sites of Cdc13, Cdc13-Myc 9 was overexpressed from pYES2-Cdc13-Myc 9 in nocodazole-arrested yeast, isolated by pull-down and SDS–PAGE and followed by the in-gel enzyme digestion. The tryptic peptides of Cdc13 were analysed by nanoscale liquid chromatography coupled to tandem mass spectrometry (nano LC-MS/MS) instrument (LTQ-FT, Thermo Fisher Scientific). The MS/MS spectra data were converted as mgf format from experiment RAW file by MM File Conversion Tools [66] ( http://www.massmatrix.net ) then analysed by MassMatrix [67] for MS/MS ion search. The search parameters in MassMatrix including the error tolerance of precursor ions and the MS/MS fragment ions in spectra were 10 p.p.m. and 0.6 Da. The enzyme for digestion was assigned to be trypsin with the miss cleavage number two. The variable post-translational modifications in search parameters were assigned to include the oxidation of methionine, carbamidomethylation of cysteine and the phosphorylation of serine/threonine/tyrosine. The phosphorylation sites of Cdc13 identified by MS were S306, T308, S314, S324, S333 and S336 ( Supplementary Fig. 10 ). In vitro kinase assay For IPs, 50 ml cultures of mid-log-phase cells were collected and lysates were prepared in 500 μl lysis buffer (100 mM NaCl, 50 mM Tris–HCl, pH 7.5, 50 mM NaF, 50 mM β-glycerophosphate, pH 7.4, 2 mM EDTA, 2 mM EGTA, 0.1% Triton X-100, 1 mM DTT and protease inhibitors) [68] . A total of 450 μl of supernatant was incubated with 50 μl protein G-coated Dynabeads (Invitrogen) and 2 μg of M2 anti-Flag antibody (Sigma) for 2 h at 4 °C. The beads were washed five times with 500 μl lysis buffer and once with 100 μl kinase buffer without ATP (50 mM Tris-HCl, pH 7.4, 1 mM DTT, 25 mM β-glycerophosphate and 5 mM MgCl 2 ) and then resuspended in buffer with 10 μM ATP, 5 μCi [ 32 P]ATP and 2 μg recombinant Cdc13(276–332) proteins for 30 min at 30 °C. Sample buffer (2 × ) was added, and reactions were separated by 10% SDS–PAGE and subjected to autoradiography using an X-ray film. Images were captured and quantified by a bioluminescence imaging system (UVP BioSpectrum AC Imagine System, UVP). Co-IP of TLC1 RNA For studies of nocodazole-arrested cell cultures, yeast cells were grown at 30 °C in complete media to OD 660 =0.8 and treated with nocodazole for 3 h. Extracts were prepared as previously described [69] . One Complete EDTA-free protease inhibitor tablet (Roche) was added for each 10 ml of TMG-50. Typically, 3 mg of total protein was adjusted to 0.5% (v/v) Tween-20 and 200 U ml −1 of RNasin (Promega) and RNaseOut (Invitrogen) before our hour incubation at 4 °C with monoclonal anti-Myc antibody (Roche). Dynabeads Protein G (Invitrogen) equilibrated with TMG-50 plus 0.5% (v/v) Tween-20 was then added and incubated for 1 h at 4 °C. Beads were washed three times with TMG-50 plus 0.5% (v/v) Tween-20, once with TMG-50 and resuspended in TMG-50. For the IP of Est1, nocodazole-arrested cells were treated with zymolyase to create spheroplasts, which were then resuspended in 1 ml lysis buffer (0.4 M sorbitol, 150 mM potassium acetate, 2 mM magnesium acetate, 20 mM HEPES/KOH, pH 6.5, 100 mg ml −1 phenylmethylsulfonyl fluoride, 1 mg ml −1 pepstatin A and 0.5 mg ml −1 leupeptin). Spheroplasts were washed three times in lysis buffer, with centrifugation at 4,200 r.p.m. for 3 min between each wash. Triton X-100 was added to 1% final concentration and the insoluble fraction was pelleted at 14,000 r.p.m. for 15 min at 4 °C (ref. 70 ). The chromatin pellet was resuspended in 1 ml TMG-50 buffer for further IP. For studies involving synchronous cultures, yeast cultures were grown at 30 °C in complete media to OD 660 =0.5. Cultures were then arrested to late G1 phase by the addition of 0.015 μg ml −1 α-factor. After arrest, α-factor was removed and cells were allowed to progress synchronously through the cell cycle at 24 °C. Samples were taken at 0, 45, 60, 70, 80 and 90 min for fluorescence-activated cell sorting and co-IP analysis. Extracts were prepared for each time point exactly as described. The amount of TLC1 and Actin mRNA copurified were quantified using real-time reverse transcription PCR; Kappa). The enrichment of TLC1 was expressed as the ratio of TLC1 amount co-immunoprecipitated in the presence of anti-Myc 9E10 antibody in samples versus lysate from untagged control strain (background) after normalization to total input ( TLC1 test IP/ TLC1 test input)( TLC1 no tag input/ TLC1 no tag). The enrichment of Actin mRNA was also calculated in the same way and used as a control. The results show an average of three experiments. Statistically significant differences in data sets were established by using a Student’s t -test. The error bars represent s.d. How to cite this article: Shen, Z.-J. et al. PP2A and Aurora differentially modify Cdc13 to promote telomerase release from telomeres at G2/M phase. Nat. Commun. 5:5312 doi: 10.1038/ncomms6312 (2014).